PAD4 regulates proliferation of multipotent haematopoietic cells by controlling c-myc expression Peptidylarginine deiminase 4 (PAD4) functions as a transcriptional coregulator by catalyzing the conversion of histone H3 arginine residues to citrulline residues. Although the high level of PAD4 expression in bone marrow cells suggests its involvement in haematopoiesis, its precise contribution remains unclear. Here we show that PAD4, which is highly expressed in lineage − Sca-1 + c-Kit + (LSK) cells of mouse bone marrow compared with other progenitor cells, controls c-myc expression by catalyzing the citrullination of histone H3 on its promoter. Furthermore, PAD4 is associated with lymphoid enhancer-binding factor 1 and histone deacetylase 1 at the upstream region of the c-myc gene. Supporting these findings, LSK cells, especially multipotent progenitors, in PAD4-deficient mice show increased proliferation in a cell-autonomous fashion compared with those in wild-type mice. Together, our results strongly suggest that PAD4 regulates the proliferation of multipotent progenitors in the bone marrow by controlling c-myc expression. Peptidylarginine deiminase (PAD/PADI, EC 3.5.3.15) is a citrullination/deimination enzyme that converts arginine residues to citrulline residues in a Ca 2+ -dependent manner [1] , [2] , [3] , [4] . There are four enzymatically active PADs (PAD1–4) that are expressed in a wide variety of tissues in humans and rodents [1] , [3] , [4] . Previously, we reported that PAD type IV (PAD4/PADI4/PADV) is localized in the nucleus and citrullinates the core histones H3, H4 and H2A, and nucleophosmin/B23 in neutrophils following calcium influx [5] , [6] . PAD4 has been recently accepted as a transcriptional coregulator. PAD4 is recruited to the promoters of genes regulated by the oestrogen receptor (ER) and p53, where it catalyzes the citrullination of the N-tail of histone H3 and inhibits arginine methylation [7] , [8] , [9] , [10] . Furthermore, on the pS2 promoter, which contains an ER response element, PAD4 interacts with histone deacetylases (HDACs) to generate a transcriptionally repressive chromatin environment [11] , [12] . More recently, it was reported that Elk-1, a member of the ETS oncogene family, is citrullinated by PAD4 to activate c-fos expression in breast cancer cells [13] . PAD4 was first identified as a protein that was induced in human promyelocytic leukaemia HL-60 cells following their differentiation into granulocytes and monocytes [14] . In mice and humans, PAD4 is expressed mainly in haematopoietic tissues such as bone marrow and spleen and also in neutrophils, eosinophils and monocytes in the peripheral blood [6] , [15] , [16] . Pathological roles for PAD4 have been reported in inflammation and chronic inflammatory diseases [17] . Various citrullinated proteins were identified as autoantigens in patients with rheumatoid arthritis [18] , [19] , [20] . Furthermore, citrullination of core histones by PAD4 in neutrophils was found to be essential for the formation of neutrophil extracellular traps induced by bacterial infections [21] , [22] . PAD inhibitors, such as Cl-amidine, have shown efficacy in animal models of rheumatoid arthritis, ulcerative colitis and cancer [23] , [24] , [25] . However, the physiological function of PAD4 in haematopoiesis remains unclear. All blood cells are generated from haematopoietic stem cells (HSCs), which reside in adult bone marrow, through several stages of myeloid and lymphoid progenitor cells. It is well known that deregulation of the proliferation and differentiation of haematopoietic progenitors causes serious diseases such as leukaemia. The proto-oncogene c-myc encodes c-myc, which has been implicated in the regulation of a wide variety of biological processes, including the control of cell division, apoptosis, cellular growth and differentiation. The expression of c-myc is strictly controlled during haematopoiesis and has important roles in the regulation of the proliferation and differentiation of HSCs and progenitor cells [26] , [27] . Lymphoid enhancer-binding factor 1 (LEF1), which acts as a transcription factor downstream of the Wnt signalling pathway, is one of the proteins involved in the regulation of c-myc expression, and its deregulation results in acute leukaemia [28] . We report here that PAD4 is expressed in bone marrow lineage − Sca-1 + c-Kit + (LSK) cells, which are primitive haematopoietic cells, and helps control c-myc expression in association with LEF1 and HDAC1. Furthermore, PAD4 deficiency causes the aberrant proliferation of LSK cells, especially multipotent progenitors (MPPs), in vivo . PAD4 expression in bone marrow LSK cells Although PAD4 is expressed in bone marrow and mature granulocytes and monocytes, its expression in haematopoietic progenitors has not been studied in detail. Initially, we performed quantitative reverse transcription–PCR (RT–qPCR) using primer sets for PAD4 and β-actin messenger RNA (mRNA) as an internal control to investigate its expression in the various stages of haematopoietic cells found in the bone marrow. The cells were sorted and collected by fluorescence-activated cell sorting (FACS) using antibodies against appropriate markers, as described in the Methods and in Supplementary Fig. S1 . RT–qPCR showed that PAD4 mRNA was expressed in Gr-1 high Mac-1 + (mature granulocytes) and Gr-1 med Mac-1 + (monocytes and immature granulocytes) cells, as previously reported, but not in B220 + B cells ( Fig. 1a ). Interestingly, PAD4 mRNA was expressed in LSK cells, which are primitive haematopoietic cells containing HSCs, MPPs, and lineage-restricted progenitors (LRPs), at a similar level to that in granulocytes ( Fig. 1a ). Furthermore, its expression in common myeloid progenitor and granulocyte-macrophage progenitor (GMP) cells was ~5-fold lower than in LSK cells, while it was barely expressed in megakaryocyte–erythrocyte progenitor cells ( Fig. 1b ). 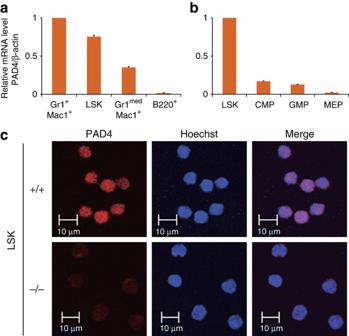Figure 1: Expression and nuclear localization of PAD4 in LSK cells. (a,b) The mRNA levels of PAD4 in various stages of haematopoietic cells. RT–qPCR analysis was performed with RNA isolated from the collected cells of (a) Gr-1highMac-1+, LSK and Gr-1medMac-1+, (b) LSK, common myeloid progenitor (CMP), GMP and megakaryocyte–erythrocyte progenitor (MEP) in the bone marrow of wild-type mice (n=3) by FACS as described in the Methods. The values were normalized to the levels of β-actin and presented as the relative level to that of (a) Gr-1highMac-1+or (b) LSK. The error bars indicate ±s.d. (c) Nuclear localization of PAD4 in LSK cells. LSK cells isolated from the bone marrow ofPADI4+/+(+/+) andPADI4−/−(−/−) mice by FACS and subjected to immunocytochemical staining with anti-PAD4 (red). The nuclei were stained with Hoechst (blue). Scale bars, 10 μm. Figure 1: Expression and nuclear localization of PAD4 in LSK cells. ( a , b ) The mRNA levels of PAD4 in various stages of haematopoietic cells. RT–qPCR analysis was performed with RNA isolated from the collected cells of ( a ) Gr-1 high Mac-1 + , LSK and Gr-1 med Mac-1 + , ( b ) LSK, common myeloid progenitor (CMP), GMP and megakaryocyte–erythrocyte progenitor (MEP) in the bone marrow of wild-type mice ( n =3) by FACS as described in the Methods. The values were normalized to the levels of β-actin and presented as the relative level to that of ( a ) Gr-1 high Mac-1 + or ( b ) LSK. The error bars indicate ±s.d. ( c ) Nuclear localization of PAD4 in LSK cells. LSK cells isolated from the bone marrow of PADI4 +/+ (+/+) and PADI4 −/− (−/−) mice by FACS and subjected to immunocytochemical staining with anti-PAD4 (red). The nuclei were stained with Hoechst (blue). Scale bars, 10 μm. Full size image Next, to analyse the expression of PAD4 protein in LSK cells, we generated an anti-mouse PAD4 monoclonal antibody (anti-PAD4). Anti-PAD4 we generated specifically recognized mouse PAD4 in immunoblotting, immunoprecipitation and immunocytochemical staining ( Supplementary Fig. S2 ). Immunocytochemical staining with anti-PAD4 showed that ~50% of mouse bone marrow cells were PAD4-positive and many of them had lobulated nuclei, which is a characteristic of mature granulocytes ( Supplementary Fig. S2c ). To examine the expression and subcellular localization of PAD4 in LSK cells, we performed immunocytochemical staining of isolated LSK cells with anti-PAD4. The results showed that specific signals were present in the nuclei of LSK cells from PADI4 +/+ mice, but not in the cells from PADI4 −/− mice ( Fig. 1c ). This finding of the high expression of PAD4 mRNA and protein in LSK cells prompted us to study the physiological role of PAD4 in these cells. PAD4 targets the c-myc promoter To investigate the role of PAD4 in LSK cells, we performed microarray analysis to assess gene expression in PADI4 −/− LSK cells compared with PADI4 +/+ LSK cells. Microarray analysis indicated that the expression level of c-myc was higher in PADI4 −/− LSK cells than in PADI4 +/+ LSK cells ( Supplementary Table S1 ). RT–qPCR also indicated that the mRNA level of c-myc in PADI4 −/− LSK cells was ~2-fold higher than in PADI4 +/+ LSK cells ( Fig. 2a ). Furthermore, western blotting showed that the protein level of c-myc in these cells was also increased by PAD4 deficiency ( Fig. 2b ). PAD4 is a transcriptional co-repressor that functions by citrullinating histone H3 and competitively suppressing arginine methylation at the promoter region of some genes [7] , [9] , [10] . Therefore, we expected that PAD4 controls c-myc transcription by the citrullination of histone H3 in the upstream region of the c-myc gene. To test this hypothesis, we performed chromatin immunoprecipitation (ChIP) analysis using LSK cells with anti-PAD4, anti-citrullinated histone H3, anti-methylated arginine histone H3 and control IgG antibodies. The precipitated DNA fragments were analysed by qPCR using primer sets for regions A, B and C in the c-myc promoter ( Fig. 2c ). PCR products for region A were clearly detected in the immunoprecipitated DNA of PADI4 +/+ cells, but not PADI4 −/− cells, with anti-PAD4 and anti-citrullinated histone H3 antibodies compared with control IgG ( Fig. 2d ), whereas regions B and C were not detected. Moreover, arginine methylation of histone H3 in this region was significantly increased in PADI4 −/− cells compared with PADI4 +/+ cells ( Fig. 2e ). 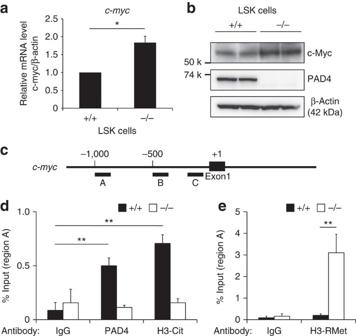Figure 2: Control of c-myc expression by PAD4 targeting toc-mycupstream. (a)c-mycmRNA levels inPADI4+/+andPADI4−/−LSK cells. LSK cells were collected by FACS fromPADI4+/+(n=3) andPADI4−/−(n=3) bone marrow and subjected to RT–qPCR. The error bars indicate ±s.d. *P=0.02. Statistical significance was determined by the standard two-tailed Student’st-test. (b) c-myc protein levels inPADI4+/+andPADI4−/−LSK cells.PADI4+/+(+/+) andPADI4−/−(−/−) LSK cells (two mice each) were analysed by western blotting with antibodies against c-myc, PAD4 and β-actin (5.0 × 104cells per lane). (c) Schematic structure of the upstream region of thec-mycgene indicating the locations of the amplified DNA (black bars: regions A, B and C) used for the ChIP assays. (d,e) ChIP assays for PAD4, citrullinated histone H3 and methylated arginine histone H3. LSK cells were collected fromPADI4+/+(black bar) (n=3) andPADI4−/−(white bar) (n=3) bone marrow cells and then subjected to the ChIP assay using control IgG (IgG), anti-PAD4 (PAD4), anti-citrullinated histone H3 (H3-Cit) and anti-methylated arginine histone H3 (H3-RMet) antibodies as described in the Methods. The error bars indicate ±s.d. **P<0.01. Statistical significance was determined by the standard two-tailed Student’st-test. Figure 2: Control of c-myc expression by PAD4 targeting to c-myc upstream. ( a ) c-myc mRNA levels in PADI4 +/+ and PADI4 −/− LSK cells. LSK cells were collected by FACS from PADI4 +/+ ( n =3) and PADI4 −/− ( n =3) bone marrow and subjected to RT–qPCR. The error bars indicate ±s.d. * P =0.02. Statistical significance was determined by the standard two-tailed Student’s t -test. ( b ) c-myc protein levels in PADI4 +/+ and PADI4 −/− LSK cells. PADI4 +/+ (+/+) and PADI4 −/− (−/−) LSK cells (two mice each) were analysed by western blotting with antibodies against c-myc, PAD4 and β-actin (5.0 × 10 4 cells per lane). ( c ) Schematic structure of the upstream region of the c-myc gene indicating the locations of the amplified DNA (black bars: regions A, B and C) used for the ChIP assays. ( d , e ) ChIP assays for PAD4, citrullinated histone H3 and methylated arginine histone H3. LSK cells were collected from PADI4 +/+ (black bar) ( n =3) and PADI4 −/− (white bar) ( n =3) bone marrow cells and then subjected to the ChIP assay using control IgG (IgG), anti-PAD4 (PAD4), anti-citrullinated histone H3 (H3-Cit) and anti-methylated arginine histone H3 (H3-RMet) antibodies as described in the Methods. The error bars indicate ±s.d. ** P <0.01. Statistical significance was determined by the standard two-tailed Student’s t -test. Full size image PAD4 is associated with a complex of LEF1 and HDAC PAD4 interacts with several transcription factors, such as p53 and ER, and functions as a transcriptional co-repressor [7] , [8] , [9] . Various transcription factors, including Rbpj, Smad1, Smad4, TCF4, STAT1, STAT4 and LEF1, are known to bind to the vicinity of region A on the c-myc promoter ( Supplementary Fig. S3a ) (ref. 29 ). These transcription factors are expressed in LSK cells ( Supplementary Fig. S3b ). To investigate whether PAD4 interacts with these transcription factors, HA-tagged PAD4 (HA-PAD4) and the FLAG-tagged transcription factors were expressed in HEK293T cells. Immunoblotting with an anti-FLAG antibody following immunoprecipitation with an anti-HA antibody showed that PAD4 interacted with LEF1, but not with the other examined transcription factors ( Fig. 3a , and Supplementary Fig. S3c ). Furthermore, immunoblotting with an anti-HA antibody following immunoprecipitation with an anti-FLAG antibody also showed this interaction ( Fig. 3a ). We observed repeatedly that PAD4 expression led to the decreased expression of Rbpj, TCF4 and STAT4 ( Supplementary Fig. S3c ). LEF1 and PAD4 reportedly interact with HDAC1 to repress the transcription of their target genes [11] , [30] . To test whether endogenous PAD4 associates with LEF1 and HDAC1, lineage − bone marrow cells were collected and then subjected to a coimmunoprecipitation assay. Immunoprecipitation with anti-PAD4 and western blotting with anti-LEF1 or anti-HDAC1 antibodies showed that endogenous LEF1 and HDAC1 coimmunoprecipitated with PAD4 ( Fig. 3b ). 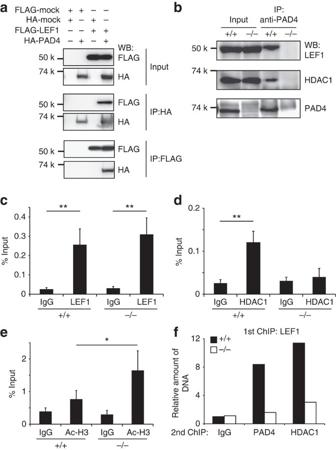Figure 3: Interaction of PAD4 with LEF1 and HDAC1. (a) Coimmunoprecipitation assays for PAD4 and LEF1 using co-transfected HEK293T cells. HEK293T cells were transfected with plasmids expressing HA-PAD4 or FLAG-LEF1, as indicated at the top. The cell lysates were immunoprecipitated with anti-HA or anti-FLAG antibodies and then subjected to western blotting of the cell lysates (input) and the immunoprecipitated proteins (IP:HA or IP:FLAG) with anti-FLAG or anti-HA antibodies, as indicated on the right. (b) Coimmunoprecipitation assays for endogenous PAD4, LEF1 and HDAC1. Lineage−cells were collected fromPADI4+/+(+/+) andPADI4−/−(−/−) bone marrow cells and then subjected to immunoprecipitation using anti-PAD4. The cell lysates (input) and the precipitated proteins (IP:anti-PAD4) were analysed by western blotting with anti-LEF1 (top), anti-HDAC1 (middle) and anti-PAD4 (bottom) antibodies. (c–e) ChIP assays for LEF1 (c), HDAC1 (d), and acetylated histone H3 (e) on thec-mycpromoter (region A). LSK cells were collected fromPADI4+/+(+/+) (n=3) andPADI4−/−(−/−) (n=3) bone marrow cells and then subjected to ChIP using control IgG, anti-LEF1 (c), anti-HDAC1 (d) and anti-acetylated histone H3 (Lys 9) (e) antibodies as described in the Methods. The error bars indicate ±s.d. **P<0.01, *P<0.05. Statistical significance was determined by the standard two-tailed Student’st-test. (f) re-ChIP assay for LEF1, PAD4 and HDAC1 on thec-mycpromoter (region A). LSK cells were collected fromPADI4+/+(black bars) andPADI4−/−(white bars) bone marrow cells and then subjected to ChIP with the anti-LEF1 antibody. The precipitated DNA–protein complexes were eluted and subjected to a second round of ChIP with control IgG, anti-PAD4 or anti-HDAC1 antibodies as described in the Methods. Figure 3: Interaction of PAD4 with LEF1 and HDAC1. ( a ) Coimmunoprecipitation assays for PAD4 and LEF1 using co-transfected HEK293T cells. HEK293T cells were transfected with plasmids expressing HA-PAD4 or FLAG-LEF1, as indicated at the top. The cell lysates were immunoprecipitated with anti-HA or anti-FLAG antibodies and then subjected to western blotting of the cell lysates (input) and the immunoprecipitated proteins (IP:HA or IP:FLAG) with anti-FLAG or anti-HA antibodies, as indicated on the right. ( b ) Coimmunoprecipitation assays for endogenous PAD4, LEF1 and HDAC1. Lineage − cells were collected from PADI4 +/+ (+/+) and PADI4 −/− (−/−) bone marrow cells and then subjected to immunoprecipitation using anti-PAD4. The cell lysates (input) and the precipitated proteins (IP:anti-PAD4) were analysed by western blotting with anti-LEF1 (top), anti-HDAC1 (middle) and anti-PAD4 (bottom) antibodies. ( c – e ) ChIP assays for LEF1 ( c ), HDAC1 ( d ), and acetylated histone H3 ( e ) on the c-myc promoter (region A). LSK cells were collected from PADI4 +/+ (+/+) ( n =3) and PADI4 −/− (−/−) ( n =3) bone marrow cells and then subjected to ChIP using control IgG, anti-LEF1 ( c ), anti-HDAC1 ( d ) and anti-acetylated histone H3 (Lys 9) ( e ) antibodies as described in the Methods. The error bars indicate ±s.d. ** P <0.01, * P <0.05. Statistical significance was determined by the standard two-tailed Student’s t -test. ( f ) re-ChIP assay for LEF1, PAD4 and HDAC1 on the c-myc promoter (region A). LSK cells were collected from PADI4 +/+ (black bars) and PADI4 −/− (white bars) bone marrow cells and then subjected to ChIP with the anti-LEF1 antibody. The precipitated DNA–protein complexes were eluted and subjected to a second round of ChIP with control IgG, anti-PAD4 or anti-HDAC1 antibodies as described in the Methods. Full size image We next examined binding of the PAD4, LEF1 and HDAC1 complexes to the c-myc promoter. A ChIP assay showed that LEF1 bound to region A on the c-myc promoter in not only PADI4 +/+ cells but also in PADI4 −/− cells ( Fig. 3c ). Conversely, HDAC1 was bound to this region in PADI4 +/+ cells, but not in PADI4 −/− LSK cells ( Fig. 3d ). In addition, the acetylation level of histone H3 (Lys 9) was slightly higher in PADI4 −/− cells than in PADI4 +/+ cells ( Fig. 3e ). To demonstrate further complex formation of PAD4 with LEF1 and HDAC1 on the c-myc promoter, we performed a re-ChIP assay. The results showed that PAD4 and HDAC1 were components of the complex that was immunoprecipitated with the anti-LEF1 antibody in PADI4 +/+ LSK cells, but not in PADI4 −/− cells ( Fig. 3f ). These results indicate that PAD4 might be required for the formation of the complex with LEF1 and HDAC1 on the c-myc promoter in LSK cells. Together, these results indicate that PAD4 targets the c-myc promoter in LSK cells in complex with LEF1 and HDAC, where histone H3 appears to be citrullinated, unmethylated and deacetylated to suppress its transcription. Proliferation of LSK cells is activated by PAD4 deficiency Next, to investigate the physiological significance of PAD4 in LSK cells in vivo , we compared the haematopoietic progenitor populations in the bone marrow of PADI4 −/− mice and their PADI4 +/+ littermates. No PAD4 protein was detected in PADI4 −/− cell lysates of bone marrow cells or LSK cells using western blotting, even in the proteins immunoprecipitated with anti-PAD4 ( Fig. 2b and Supplementary Fig. S2c ). FACS analysis showed that the percentage of LSK cells in PADI4 −/− mice was higher than in PADI4 +/+ mice ( Fig. 4a ), while the populations of myeloid progenitor cells (common myeloid progenitor, GMP and megakaryocyte–erythrocyte progenitor cells) were not affected significantly by PAD4 deficiency ( Supplementary Fig. S5a ). To analyse the proliferation state of LSK cells, we performed an in vivo 5-bromo 2'-deoxyuridine (BrdU)-incorporation assay. After the injection of BrdU, we analysed the ratio of BrdU-positive LSK cells in the bone marrow. FACS analysis showed that the ratio of BrdU-incorporated LSK cells in PADI4 −/− mice was higher than in PADI4 +/+ mice, suggesting that the proliferation of LSK cells was activated by PAD4 deficiency ( Fig. 4c ). The proliferation of LSK cells is strictly regulated by intracellular signals, as well as the microenvironment of the bone marrow. To examine whether the increased proliferation of LSK cells by PAD4 deficiency was caused by a cell-autonomous effect, we performed bone marrow transplantation (BMT) using C57BL/6-Ly-5.1 mice (B6/Ly-5.1), which are a B6 background congenic strain with a differential B cell antigen designated as Ly-5.1 ( Fig. 4e ). The percentage of LSK cells in PADI4 −/− BMT recipient mice from B6/Ly-5.1 donor mice was similar to that in PADI4 +/+ recipient mice ( Fig. 4e ). Conversely, the percentage of LSK cells in B6/Ly-5.1 BMT recipient mice from PADI4 −/− donor mice was higher than in B6/Ly-5.1 recipient mice from PADI4 +/+ donor mice ( Fig. 4f ). These results indicate that the increased proliferation of PADI4 −/− LSK cells in the bone marrow proceeds in a cell-autonomous fashion, suggesting that the elevated expression of c-myc by PAD4 deficiency results in the higher proliferation rate of these cells. 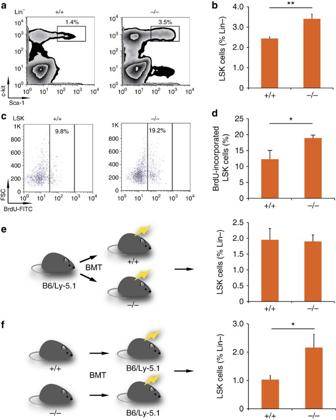Figure 4: Increased proliferation of LSK cells inPADI4−/−mice in a cell-autonomous fashion. (a) Representative FACS results for the proportion of LSK cells inPADI4+/+andPADI4−/−mice. Bone marrow cells fromPADI4+/+(+/+) andPADI4−/−(−/−) mice were stained with the antibodies against lineage-FITC, c-Kit-APC and Sca-1-PE and analysed by FACS. LSK cells were gated by the square and shown as their percentage of the lineage−cells. (b) The histograms show the average percentage of LSK cells inPADI4+/+(+/+) (n=7) andPADI4−/−(−/−) (n=7) mice. The error bars indicate ±s.e.m. **P=0.002. Statistical significance was determined by the standard two-tailed Student’st-test. (c) Representative results of BrdU-incorporated LSK cells. BrdU-incorporated LSK cells were analysed by FACS as described in the Methods. (d) The histograms show the average percentage of BrdU-positive LSK cells inPADI4+/+(+/+) (n=3) andPADI4−/−(−/−) mice (n=3). The error bars indicate ±s.e.m. *P=0.04. Statistical significance was determined by the standard two-tailed Student’st-test. (e,f) Scheme of the BMT assay and the percentage of LSK cells in the BMT recipients. The proportion of LSK cells were analysed by FACS after BMT of (e)PADI4+/+(+/+) (n=5) orPADI4−/−(−/−) (n=6) recipients from B6/Ly5.1 donors and (f) B6/Ly5.1 recipients (n=5 for each donor) fromPADI4+/+(+/+) orPADI4−/−(−/−) donors. The histograms show the average percentage of LSK cells in the bone marrow of the recipients. The error bars indicate ±s.e.m. *P=0.03. Statistical significance was determined by the standard two-tailed Student’st-test. Figure 4: Increased proliferation of LSK cells in PADI4 −/− mice in a cell-autonomous fashion. ( a ) Representative FACS results for the proportion of LSK cells in PADI4 +/+ and PADI4 −/− mice. Bone marrow cells from PADI4 +/+ (+/+) and PADI4 −/− (−/−) mice were stained with the antibodies against lineage-FITC, c-Kit-APC and Sca-1-PE and analysed by FACS. LSK cells were gated by the square and shown as their percentage of the lineage − cells. ( b ) The histograms show the average percentage of LSK cells in PADI4 +/+ (+/+) ( n =7) and PADI4 −/− (−/−) ( n =7) mice. The error bars indicate ±s.e.m. ** P =0.002. Statistical significance was determined by the standard two-tailed Student’s t -test. ( c ) Representative results of BrdU-incorporated LSK cells. BrdU-incorporated LSK cells were analysed by FACS as described in the Methods. ( d ) The histograms show the average percentage of BrdU-positive LSK cells in PADI4 +/+ (+/+) ( n =3) and PADI4 −/− (−/−) mice ( n =3). The error bars indicate ±s.e.m. * P =0.04. Statistical significance was determined by the standard two-tailed Student’s t -test. ( e , f ) Scheme of the BMT assay and the percentage of LSK cells in the BMT recipients. The proportion of LSK cells were analysed by FACS after BMT of ( e ) PADI4 +/+ (+/+) ( n =5) or PADI4 −/− (−/−) ( n =6) recipients from B6/Ly5.1 donors and ( f ) B6/Ly5.1 recipients ( n =5 for each donor) from PADI4 +/+ (+/+) or PADI4 −/− (−/−) donors. The histograms show the average percentage of LSK cells in the bone marrow of the recipients. The error bars indicate ±s.e.m. * P =0.03. Statistical significance was determined by the standard two-tailed Student’s t -test. Full size image Number of MPPs in LSK cells is increased by PAD4 deficiency It is known that the LSK population contains at least three cell types—HSCs, MPPs and LRPs—and each can be determined as CD150 + CD48 − , CD150 − CD48 − and CD150 − CD48 + cells, respectively [31] . To reveal which cell type was affected in the LSK population by PAD4 deficiency, bone marrow cells taken from a femur of PADI4 +/+ and PADI4 −/− mice were analysed by FACS to calculate the number of each type of cell ( Fig. 5a ). The number of LSK cells was higher in PADI4 −/− mice than in PADI4 +/+ mice, suggesting that the increased proportion of LSK cells shown in Fig. 4 was caused by an increase in their number. In the LSK population, the number of MPPs, but not HSCs or LRPs, was significantly higher in PADI4 −/− mice than in PADI4 +/+ mice ( Fig. 5b ). Furthermore, the expression level of PAD4 mRNA was highest in MPPs among these three types of cell ( Fig. 5c ). Thus, MPPs in the LSK population were affected mainly by PAD4 deficiency. 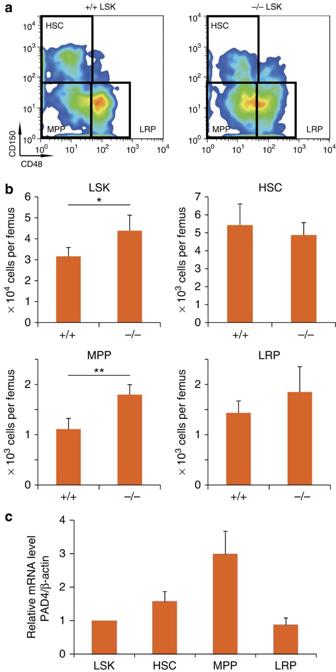Figure 5: Increased absolute number of MPPs inPADI4−/−LSK cells. (a) Representative FACS results for the proportion of HSCs, MPPs and LRPs inPADI4+/+andPADI4−/−mice. Bone marrow cells fromPADI4+/+(+/+) andPADI4−/−(−/−) mice were stained with the antibodies against lineage-FITC, c-Kit-PerCP, Sca-1-PE, CD48-biotin, CD150-APC and streptavidin-eFluoro 450 and analysed by FACS. HSCs, MPPs and LRPs were determined as CD150+CD48−, CD150−CD48−and CD150−CD48+cells, respectively. (b) The histograms show the average number of LSK cells, HSCs, MPPs and LRPs in a femur fromPADI4+/+(+/+) (n=6) andPADI4−/−(−/−) (n=8) mice. The error bars indicate ±s.d. *P<0.05, **P<0.01. Statistical significance was determined by the standard two-tailed Student’st-test. (c) Expression of PAD4 mRNA in HSCs, MPPs and LRPs. RT–qPCR analysis was performed with RNA isolated from LSK cells, HSCs, MPPs and LRPs collected from the bone marrow of wild-type mice (n=3) by FACS. The values were normalized to the levels of β-actin and presented as the relative level to that of LSK. The error bars indicate ±s.d. Figure 5: Increased absolute number of MPPs in PADI4 −/− LSK cells. ( a ) Representative FACS results for the proportion of HSCs, MPPs and LRPs in PADI4 +/+ and PADI4 −/− mice. Bone marrow cells from PADI4 +/+ (+/+) and PADI4 −/− (−/−) mice were stained with the antibodies against lineage-FITC, c-Kit-PerCP, Sca-1-PE, CD48-biotin, CD150-APC and streptavidin-eFluoro 450 and analysed by FACS. HSCs, MPPs and LRPs were determined as CD150 + CD48 − , CD150 − CD48 − and CD150 − CD48 + cells, respectively. ( b ) The histograms show the average number of LSK cells, HSCs, MPPs and LRPs in a femur from PADI4 +/+ (+/+) ( n =6) and PADI4 −/− (−/−) ( n =8) mice. The error bars indicate ±s.d. * P <0.05, ** P <0.01. Statistical significance was determined by the standard two-tailed Student’s t -test. ( c ) Expression of PAD4 mRNA in HSCs, MPPs and LRPs. RT–qPCR analysis was performed with RNA isolated from LSK cells, HSCs, MPPs and LRPs collected from the bone marrow of wild-type mice ( n =3) by FACS. The values were normalized to the levels of β-actin and presented as the relative level to that of LSK. The error bars indicate ±s.d. Full size image In this study, we presented a new role for PAD4 in the regulation of the proliferation of bone marrow LSK cells. Our results indicated that PAD4 appears to be involved in the control of c-myc transcription in LSK cells by histone citrullination and antagonizing arginine methylation. A previous report using genome-wide analysis with a ChIP-coupled chip showed that PAD4 binds to the upstream region of c-myc [13] . The expression of c-myc in LSK cells was regulated by not only transcriptional but also post-transcriptional events that are important for the maintenance of LSK cells [32] . Both the protein and mRNA levels of c-myc in PADI4 −/− LSK cells were increased compared with PADI4 +/+ LSK cells, suggesting that transcriptional regulation may be crucial for controlling c-myc expression. The microarray analysis revealed several genes involved in cell proliferation showed difference in expression between PADI4 −/− and PADI4 +/+ LSK cells although c-myc is at least one of the important target genes involved in PAD4-dependent proliferation regulation of LSK cells. Further experiments are requisite to assess whether other genes whose expression was different in PADI4 −/− and PADI4 +/+ LSK cells are involved in PAD4-dependent regulation of LSK proliferation. We found that PAD4 associates with LEF1 and HDAC1, binds to the upstream region of the c-myc gene, and may function as a repressor complex. Our results from the ChIP assay indicated that arginine methylation of histone H3 on the c-myc promoter was increased in the absence of PAD4. Several groups have suggested that PAD4 can convert methylarginine to citrulline in histone H3, whereas others have demonstrated that PAD4 does not possess physiologically relevant activity in vitro [33] . The citrullination of arginine residues by PAD4 might make it impossible for arginine methyltransferases to methylate them in MPP cells. We showed that HDAC1 did not bind to the LEF1-PAD4-binding region of the c-myc promoter in PADI4 −/− cells and that the acetylation of histone H3 was slightly increased. This suggests that not only increased arginine methylation but also acetylation of histone H3 might lead to the activation of c-myc transcription in PADI4 −/− cells. Neither HDAC1 nor PAD4 was detected in regions B or C of the c-myc promoter, whereas acetylated histone H3 (Lys 9) was detected at region C and the acetylation level there was comparable between PAD4 +/+ and PAD4 −/− cells ( Supplementary Fig. S4a ). In addition, loading of RNA polymerase II to the transcriptional start site of the c-myc gene was not changed in PADI4 −/− cells ( Supplementary Fig. S4b ). Further study is necessary to elucidate fully the molecular mechanisms underlying the transcriptional regulation of c-myc by histone citrullination. LEF1 represses the transcription of its target genes by recruiting an HDAC1-containing co-repressor complex, while the binding of β-catenin, which acts downstream of the Wnt signalling pathway, to LEF1 leads to the release of HDAC1, resulting in transcriptional activation [30] . Although this mechanism might be involved in the activation of c-myc transcription in LSK cells, histone H3 citrullination was maintained because the reverse conversion of citrullination was not found. Additional modifications, such as acetylation, might be required for the transactivation of the transcription repressed by histone citrullination. The Wnt signalling pathway plays crucial roles in the regulation of stem cell fate in various tissues, including HSCs [34] , [35] , [36] . As the balance between the self-renewal and differentiation of haematopoietic stem/progenitor cells is controlled precisely by various soluble factors, cell–cell communications, and intracellular signals in their microenvironment, PAD4 may be involved in their regulation. Although one of the major target genes for LEF1 is the c-myc oncogene, PAD4 might act as a co-repressor for not only c-myc but also other targets of LEF1. We demonstrated the expression of PAD4 in LSK cells of the bone marrow by using RT–qPCR and immunocytochemical staining. The RT–qPCR results showed that PAD4 mRNA levels in myeloid progenitors were much lower than in granulocytes and LSK cells. This result is consistent with the induction of PAD4 expression during the differentiation of HL-60 cells, corresponding to the stage of GMP cells, into granulocytes [14] . The observation that the proportion of mature granulocytes (Gr-1 high Mac-1 + ) in bone marrow was not affected in PADI4 −/− mice ( Supplementary Fig. S5b ) may suggest that PAD4 is not essential for their differentiation. Interestingly, PAD4 expression appeared to be downregulated during the maturation of HSCs into myeloid progenitors and then upregulated during the maturation of GMP cells into granulocytes or monocytes. Although the regulation of PAD4 transcription by ER and p53 in MCF-7 and U373MG cells, respectively, has been reported [37] , [38] , the controlling mechanisms for PAD4 expression during haematopoiesis remain to be studied. We showed here that PAD4 is one of the suppressive regulators of proliferation in LSK cells, especially MPP cells, by controlling c-myc expression, suggesting that PAD4 may function as a tumour suppressor. In fact, the ectopic expression of PAD4 in A549, U2OS and HCT116 cancer cells suppresses their proliferation [38] . In addition, the crucial role of PAD4 in histone H4 citrullination for the induction of apoptosis in response to DNA damage has been published [39] . Conversely, the inhibition of PAD4 activity in U2OS cells using a PAD4 inhibitor (Cl-amidine) or siRNA reportedly suppresses cell proliferation [9] , [25] , [40] . The effect of PAD4 activity on cell proliferation might depend on cell type, signalling pathway for its activation, and its substrate proteins. The overexpression of PAD4 in the M1 mouse leukaemia cell line did not affect c-myc expression; however, IL-6 treatment, which can induce differentiation of these cells, caused a more efficient reduction of c-myc expression in PAD4-expressing cells than in the parent cells (unpublished data, K.N.). This suggests that a signalling pathway for PAD4 activation might be required for the regulation of c-myc expression by PAD4. PAD4 is one of the most downregulated genes in myeloid progenitor cells in MLL-rearranged leukaemia [41] ; however, we did not observe spontaneous leukemogenesis in PADI4 −/− mice or recipient mice of PADI4 −/− bone marrow, despite performing a second serial BMT. Although these findings indicate that PAD4 deficiency is unable to initiate leukemogenesis, it might be involved in the pathogenesis of some myeloproliferative diseases. Mice PADI4 −/− mice were generated by replacing exon 1 and 2, including the transcription initiation site to neomycine resistant gene as described previously [39] . All PADI4 −/− mice used in this study were backcrossed for 10 generations into the C57BL/6 background. C57BL/6-Ly-5.1 mice were obtained from the RIKEN BioResource Center. All mice were maintained in a specific pathogen-free environment and used at the age of 7–10 weeks. All animal experiments, except the generation of the monoclonal antibody (see below), were approved by the Committee for Ethics in Animal Experiments of the University of Tokyo and carried out under the Guidelines for Animal Experiments of the University of Tokyo. Cell culture and transfection HEK293T cells were cultured in DMEM supplemented with 10% fetal bovine serum and gentamicin (Life Technologies) at 37 °C in 5% CO 2 . HEK293T cells were transfected with expression plasmids using X-tremeGENE 9 (Roche) according to the manufacturer’s instructions. Preparation of the anti-mouse PAD4 monoclonal antibody Recombinant mouse PAD4 tagged with glutathione S -transferase (GST) (GST-mPAD4) was purified from Escherichia coli using a slightly modified GST-hPAD4 purification method to that described previously [14] . Briefly, E. coli transformed with pGEX-mPAD4 were cultured in 2 × YT medium, and its expression was induced by isopropyl-β- D -thiogalactoside at 25 °C for 16 h. E. coli were extracted in a lysis buffer (50 mM Tris-HCl, pH 8.0, 200 mM NaCl, 10% glycerol, 1 mM EDTA, 1 mM dithiothreitol and 1 mM phenylmethylsulfonyl fluoride) and GST-mPADI4 was purified from the extract using glutathione Sepharose 4B (GE Healthcare). To generate anti-PAD4, we immunized mice with recombinant GST-mPAD4, and serum titres were monitored by immunoblotting using lysates of mouse bone marrow cells. Clonal populations of fusion cells were screened using enzyme-linked immunosorbent assays for antibody production against recombinant mPAD4 and GST. Productive cells were cloned to monoclonal lines by serial dilution screening. Highly concentrated monoclonal antibodies were isolated from murine ascites after an intraperitoneal injection of hybridoma cells. Antibody generation conformed to the guidelines outlined in the Guide for the Care and Use of Laboratory Animals of Japan and were approved by the Animal Care Committee of Shimane University. FACS and cell sorting The following monoclonal antibodies were used for flow cytometry and cell sorting: CD150 (1:100; TC15-12F12.2), CD48 (1:100; HM48-1) c-Kit (1:200; 2B8), Sca-1 (1:200; D7), FcγR (1:100; 93), CD34 (1:100; RAM34), Ly5.1 (1:200; A20), Ly5.2 (1:200; 104), CD3e (1:200; 145-2C11), B220 (1:300; RA3-6B2), TER-119 (1:200; TER-119), Gr-1 (1:200; RB6-8C5), and Mac-1 (1:200; M1/70). A mixture of monoclonal antibodies recognizing CD3, B220, TER-119, Mac-1 or Gr-1 was used to identify lineage + cells. All monoclonal antibodies were from BD Biosciences or eBioscience. Flow cytometry was carried out on an LSR II. Cell sorting was performed on a FACS Aria II. Quantitative reverse transcription–PCR Total RNA (0.5 μg) isolated using TRIzol (Life Technologies) was reverse-transcribed with SuperScript III (Life Technologies) using random primers. The synthesized complementary DNA (cDNA) was used as a template for qPCR using Power SYBR Green Master Mix (Life Technologies) on an Applied Biosystems 7500Fast (Life Technologies). The primer sequences are presented in Supplementary Table S2 . The relative expression level was calculated by the ΔΔCt method using β-actin as an internal control. All experiments were performed in duplicate wells and with more than three independent samples. Microarray analysis Cy3-labelled antisense RNA (cRNA) was synthesized from 300 ng total RNA with a One-Color Agilent Quick Amp labeling kit (Agilent Technologies). After checking the quality and quantity of cRNA, the cRNA was allowed to hybridize at 65 °C for 17 h to an Agilent Whole-Mouse Genome Microarray 4 × 44 K. After washing, microarrays were scanned on an Agilent DNA microarray scanner (G2565BA) using one-colour scan setting. All procedures from labelling to scanning were performed according to the manufacturer’s protocols. The intensity value of each scanned feature was quantified with Agilent Feature Extraction Software v9.5 (Agilent Technologies), which performs background subtractions. Data normalization was performed by a 75 percentile median shift method. Immunocytochemical staining Bone marrow cells and isolated LSK cells were fixed with 4% paraformaldehyde and cytospun onto glass slides. The cells were heated in a 20 mM citrate buffer (pH 6.0) in a microwave oven and then stained with anti-PAD4 (1 μg ml −1 ). The antibody was probed with a goat anti-mouse antibody conjugated with Alexa Fluor 594 (1:500; Life Technologies) and the nuclei were stained with Hoechst. The signals were visualized under an LSM510 confocal microscope (Carl Zeiss). ChIP and re-ChIP assays The ChIP assays were performed using a LowCell ChIP Kit (Diagenode) according to the manufacturer’s instructions. Briefly, LSK cells (1.0 × 10 5 cells) obtained from bone marrow by FACS were fixed with 1% formaldehyde and extracted in an extraction buffer. Cross-linked chromatin was sonicated using an Ultrasonic Processor GE130 at five cycles of a 1-min pulse at 40% power with a 1-min interval between cycles. Chromatin isolated from 1.0 × 10 4 cells was used for immunoprecipitation with each antibody. For immunoprecipitation, 1 μg mouse IgG (Sigma) as a negative control, anti-PAD4 (1 μg), anti-citrullinated histone H3 (citrulline 2+8+17) (Abcam) (1 μg), anti-methylated arginine histone H3 (asymmetric dimethyl R17) (Abcam) (1 μg), anti-acetylated histone H3 (Lys 9) (Abcam) (1 μg), anti-RNA polymerase II (4H8) (Cell Signaling Technology) (1 μg), anti-LEF1 (C12A5) (Merck) (5 μl), and anti-HDAC1 (10E2) (Abcam) (5 μl) antibodies were used. The cell extracts were immunoprecipitated using the antibody-bound protein G magnetic beads and the beads were then washed. The precipitated DNA was incubated with proteinase K and then boiled for 15 min to isolate the DNA. The eluted DNA was analysed by qPCR as described above, and Ct values were used to calculate the percentage of input enrichment. For the re-ChIP assay, 1.0 × 10 6 cells were used for the initial ChIP with the anti-LEF1 antibody (10 μg) as described above. After washing the beads, protein–DNA complexes were eluted with 15 μl of 10 mM dithiothreitol at 37 °C for 30 min. The eluted solution was diluted with 1 ml ChIP buffer and then subjected to a second round of ChIP according to the ChIP protocol described above. The primer sequences are presented in Supplementary Table S1 . Plasmids and cDNA cloning Expression plasmids for FLAG-tagged transcription factors and HA-tagged PAD4 were constructed using pFLAG-CMV-2 (Sigma) and pcDNA3.1 (Invitrogen), respectively. The cDNAs of the transcription factors and PAD4 were cloned by PCR using KOD-Plus Taq DNA polymerase (TOYOBO) with the primer sets presented in Supplementary Table S2 . Immunoprecipitation and immunoblotting The cells were lysed in TSE buffer (50 mM Tris-HCl, pH 8.0, 200 mM KCl, 2 mM EDTA and 0.4% NP-40) containing a protease inhibitor cocktail (Roche) on ice for 30 min. The cell lysate was centrifuged at 15,000 g for 10 min and the supernatant was then subjected to immunoprecipitation. For co-transfected cells, the cell extracts were immunoprecipitated using an anti-HA affinity matrix (Roche) or anti-FLAG M2 agarose (Sigma) and washed five times with TSE buffer. The precipitated proteins were eluted with Laemmli sample buffer and then subjected to western blotting with anti-HA (1:2,500; Roche; 3F10) or anti-FLAG (1:2,000; Sigma) antibodies conjugated with horseradish peroxidase. For endogenous PAD4, the cell extract was incubated with 5 μg anti-PAD4 for 16 h at 4 °C and then precipitated with protein G Sepharose (Sigma). The precipitated proteins were eluted with Laemmli sample buffer and then subjected to western blotting with anti-LEF1 (1 μg ml −1 ; Millipore; #17-064), anti-HDAC1 (1:500; Abcam; 10E2), or anti-PAD4 (1 μg ml −1 ) as primary antibodies. The antibodies were probed with an anti-mouse IgG, light chain-specific (Jackson ImmunoResearch), antibody conjugated with horseradish peroxidase. Bone marrow transplantation Bone marrow cells (2.0 × 10 6 cells) taken from donor femur and tibial bones were injected intravenously in lethally irradiated (9.5 Gy) recipient mice. After 2 months, 85–90% of peripheral B220 + cells in the recipient mice were replaced with donor cells. In vivo BrdU-incorporation assay BrdU (2 mg; BD Bioscience) was injected into the abdominal cavity of the mice. After 24 h, bone marrow cells were taken from the femur and stained with the antibodies for FACS, lineage-PE, Sca-1-PerCP and c-Kit-APC, as described above. After staining, the cells were fixed with the Cytofix/Cytoperm solution (BD Bioscience) and then treated with phosphate-buffered saline containing 0.1% Triton X-100 for 10 min on ice. The cells were fixed again with the Cytofix/Cytoperm solution and treated with 300 μg ml −1 DNa se I at 37 °C for 1 h. The cells were stained with an anti-BrdU antibody conjugated with FITC and subjected to FACS analysis. Statistical analysis Data were analysed using the two-tailed unpaired Student’s t -test. All data are reported as mean±s.e.m. or s.d. Statistical analysis was performed using Excel software. Accession codes: The microarray data have been deposited to NCBI’s Gene Expression Omnibus with accession number GSE45482 . How to cite this article: Nakashima, K. et al . PAD4 regulates proliferation of multipotent haematopoietic cells by controlling c-myc expression. Nat. Commun. 4:1836 doi: 10.1038/ncomms2862 (2013).